Experimental realization of photonic topological insulator in a uniaxial metacrystal waveguide Photonic analogue of topological insulator was recently predicted by arranging ε/μ (permittivity/permeability)-matched bianisotropic metamaterials into two-dimensional superlattices. However, the experimental observation of such photonic topological insulator is challenging as bianisotropic metamaterial is usually highly dispersive, so that the ε/μ -matching condition can only be satisfied in a narrow frequency range. Here we experimentally realize a photonic topological insulator by embedding non-bianisotropic and non-resonant metacrystal into a waveguide. The cross coupling between transverse electric and transverse magnetic modes exists in metacrystal waveguide. Using this approach, the ε/μ -matching condition is satisfied in a broad frequency range which facilitates experimental observation. The topologically non-trivial bandgap is confirmed by experimentally measured transmission spectra and calculated non-zero spin Chern numbers. Gapless spin-filtered edge states are demonstrated experimentally by measuring the magnitude and phase of the fields. The transport robustness of the edge states is also observed when an obstacle was introduced near the edge. A signature of a topological state [1] , [2] , [3] , [4] , [5] , [6] , [7] , [8] , [9] is the presence of a topologically protected-edge state, resulting in a quantized conductance. Intense efforts have been devoted to realize analogous robust states in photonic systems [10] . For example, a chirality-based robust transport was first observed in time-reversal (TR) invariant photonic crystals [11] that are topologically ‘trivial’. Non-trivial bandgap characterized by non-zero Chern numbers has been achieved in TR broken photonic systems with either external magnetic field [12] , [13] , [14] , [15] or dynamical modulation [16] . Coupled helical waveguide array [17] and hyperbolic metamaterial [18] were utilized to explore topological state by breaking z -reversal symmetry. In addition, topological state associated with Weyl point has also been mapped to photonic system [19] . TR-invariant topological state of quantum spin Hall insulator has been mapped to photonic systems using two approaches, namely coupled resonator optical waveguides (CROW) [20] , [21] , [22] and bianisotropic metacrystals [23] . The CROW approach employs the resonant modes to realize pseudo-spin states and topological edge states in such system was observed in optical regime very recently [21] . As the CROW approach utilizes the resonances of ring resonators, the bandwidth of the non-trivial bandgap is inherently narrow. In the bianisotropic metacrystal approach [23] , pseudo-spin-up/spin-down states are formed using the in-phase/out-of-phase transverse electric (TE)–transverse magnetic (TM) coupled waves in a metacrystal in which the permittivity and permeability are tuned to be equal. This approach can potentially provide a somewhat broader bandwidth, but the challenge for experimental realization is the intrinsically weak bianisotropic coupling in metamaterials [24] , [25] . In this paper, we experimentally realize photonic topological insulator (PTI) using a scheme inspired by the second approach, but instead of using bianisotropic coupling, we introduce a strong effective coupling by employing ‘symmetry reduction’, which naturally couples TE/TM modes. TE and TM modes are eigensolutions in a two-dimensional configuration (invariant in the z direction) but when confined to a waveguide, these modes couple naturally and the coupling can be strong. Moreover, we use non-resonant elements [26] , [27] , [28] so that the PTI possesses large topological non-trivial bandgap and the topological edge states cover a larger frequency range. Effective bianisotropy in metacrystal waveguide Consider a spin-degenerate uniaxial medium with and sandwiched by two perfect electric conductor (PEC) plates at z =0 and z = d . We assume that the permittivity and permeability tensors are the functions of ( x,y ), but invariant in the z direction. The ratio is a constant in the whole space. Then, the Maxwell equations have the form of: For the m-th order modes in PEC waveguide, we have: where e x , e y , e z , h x , h y and h z are the functions of ( x,y ) only. For compactness, we express them in this form, and . This form automatically satisfies the PEC boundary conditions. Equation (1) can be rewritten as: where is an effective magnetoelectric coefficient tensor, with the non-zero elements of for m ≠0. Denoting a vector , we can establish a pair of decoupled spin-polarized states (spin-up) and (spin-down) that are linked by TR symmetry. Equation (3) can be rewritten in terms of , These are the two equations for wave functions of a non-relativistic particle in opposite vector potentials but same scalar potentials (see more detail in Supplementary Note 2 ). A PEC waveguide filled with spin-degenerate uniaxial medium could be mapped to a photonic quantum spin Hall system that is effectively two copies of quantum Hall systems, when the non-zero order mode is considered. The permittivity and permeability tensors are spatially dependent, and one may construct a PTI using a periodic array of non-bianisotropic cylinders constructed by non-resonant meta-atom ( Fig. 1c–f ) in the experiment. In addition, wave propagation in bianisotropic media can also be comprehended through the solution on magnetic medium (see Supplementary Fig. 1 and Note 1 ). 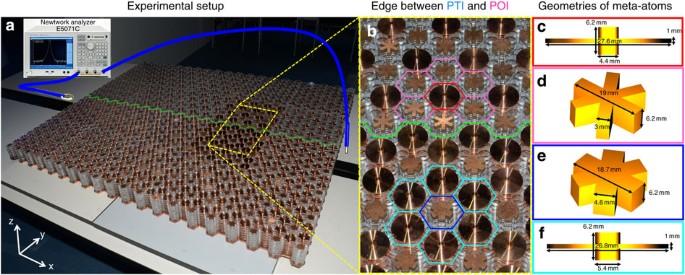Figure 1: PTI and POI. Both insulators are waveguides filled with hexagonal metacrystals. (a) Photograph of two experimental samples with the top copper plate removed to show the geometry inside. Spin-filtered EM waves are guided at the edge (green line) between both insulators. (b) Zoom-in near the edge. The hexagonal unit cells of PTI (blue and cyan hexagons) and POI (pink and red hexagons) are composed of ‘gyro’ and ‘star’ non-resonant meta-atoms. (c,d) Geometry dimensions for POI. (e,f) Geometry dimensions for PTI. Figure 1: PTI and POI. Both insulators are waveguides filled with hexagonal metacrystals. ( a ) Photograph of two experimental samples with the top copper plate removed to show the geometry inside. Spin-filtered EM waves are guided at the edge (green line) between both insulators. ( b ) Zoom-in near the edge. The hexagonal unit cells of PTI (blue and cyan hexagons) and POI (pink and red hexagons) are composed of ‘gyro’ and ‘star’ non-resonant meta-atoms. ( c , d ) Geometry dimensions for POI. ( e , f ) Geometry dimensions for PTI. Full size image Topological phases in conceptual metacrystal waveguides Consider a hexagonal metacrystal waveguide with a three-dimensional unit cell (inset of Fig. 2a ). The rod (solid) is surrounded by the background material (translucent). The rod has a hexagonal cross-section with the size of a . The lattice constant and the height of waveguide are and 1.6 a , respectively. 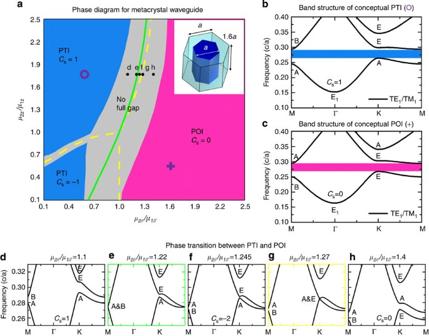Figure 2: Non-trivial/trivial bandgaps in the conceptual metacrystal waveguide design. A hexagonal lattice of anisotropic rods is embedded in a PEC waveguide. The field inhomogeneities give rise to the cross coupling between TE1and TM1modes and open a topologically non-trivial bandgap. (a) Phase diagram for the lowest bandgap. Blue and red regions indicate the non-trivial and trivial complete gap, and grey region represents the partial gap. The solid and dashed curves show the mode exchange at M and K-points. The transition between PTI and POI coincides with a gap reopening and mode exchanges at M and K points, due to the different topologies of two insulators. (b) Band structure of PTI. The constitutive parameters correspond to the purple open circle inawith the value ofε2=13μ2,μ2=diag{0.39, 0.39, 0.44} in the rod andε1=13μ1,μ1=diag{0.67, 0.67, 0.25} in the background. (c) Trivial band structure of POI. The constitutive parameters correspond to the purple cross in (a) with the value of ε2=13μ2, μ2=diag{0.72, 0.72, 0.22},ε1=13μ1andμ1=diag{0.45, 0.45, 0.41}. (d–h) Band structures in the transition region between PTI and POI phase that correspond to the black points ina. The irreducible representations of the eigenmodes are marked to see the band inversion. Figure 2b is the band structure for the first order ( m =1) modes of a topologically non-trivial metacrystal waveguide. All the bands are doubly spin-degenerate because of ε / μ -matching and inversion symmetry. Note that breaking inversion symmetry will lift the spin degeneracy at all the k-points except TR-invariant points. But this should not affect the existence of topological phases and corresponding robust edge states, as long as the bandgap does not close. A complete bandgap exists from 0.264 to 0.293 ( c / a ; blue in Fig. 2b ). Although zero order modes are also allowed in the frequency range, they would not couple to other order modes because of orthogonality. Figure 2: Non-trivial/trivial bandgaps in the conceptual metacrystal waveguide design. A hexagonal lattice of anisotropic rods is embedded in a PEC waveguide. The field inhomogeneities give rise to the cross coupling between TE 1 and TM 1 modes and open a topologically non-trivial bandgap. ( a ) Phase diagram for the lowest bandgap. Blue and red regions indicate the non-trivial and trivial complete gap, and grey region represents the partial gap. The solid and dashed curves show the mode exchange at M and K-points. The transition between PTI and POI coincides with a gap reopening and mode exchanges at M and K points, due to the different topologies of two insulators. ( b ) Band structure of PTI. The constitutive parameters correspond to the purple open circle in a with the value of ε 2 =13 μ 2 , μ 2 =diag{0.39, 0.39, 0.44} in the rod and ε 1 =13 μ 1 , μ 1 =diag{0.67, 0.67, 0.25} in the background. ( c ) Trivial band structure of POI. The constitutive parameters correspond to the purple cross in ( a ) with the value of ε 2 =13μ 2 , μ 2 = diag {0.72, 0.72, 0.22}, ε 1 =13 μ 1 and μ 1 =diag{0.45, 0.45, 0.41}. ( d – h ) Band structures in the transition region between PTI and POI phase that correspond to the black points in a . The irreducible representations of the eigenmodes are marked to see the band inversion. Full size image The spin Chern number is the topological invariant to characterize the non-trivial feature. It can be calculated by either integrating the Berry curvature over the Brillion zone [22] or analysing the symmetry of the lowest band at high symmetry k-points [29] . A non-zero spin Chern number of the band implies a non-trivial bandgap above that band. Gapless robust edge states can be predicted in the bandgap to appear at the edge of this metacrystal waveguide (see Supplementary Figs 2, 3 and Note 3 ). The bandgap can be tuned to be either topologically non-trivial or trivial, depending on the constitutive parameters of anisotropic media. Figure 2a is a phase diagram of the bandgap. The ratio μ 1 z / μ 1// is set to be 1. This ratio mainly affects the cutoff frequency at Γ point and the midgap frequency, but not the salient features of the phase diagram shown in Fig. 2a . The grey area, representing the absence of a complete bandgap, partitions the phase diagram into three regions with either trivial or non-trivial bandgap. Figure 2c shows the band structure with the complete bandgap marked with magenta color for a configuration corresponding to a photonic ordinary insulator (POI), which has identical geometry as PTI except the constitutive parameters corresponds to the purple cross in Fig. 2a . The POI has a zero spin Chern number. It possesses a trivial phase and the gapped edge states will appear (see Supplementary Fig. 3 and Note 3 ). Because of the topological character, each phase in the diagram is an isolated ‘island’. The non-trivial phase cannot be adiabatically connected to a trivial phase without closing and reopening the bandgap. The green solid line (yellow dashed line) in Fig. 2a highlights the band inversion at M (K) point. Two pairs of modes at M (K) point exchange their positions, involving the bandgap’s closing and reopening. The spin Chern number changes together with the topological phase. To show the band inversion between non-trivial and trivial phases, Fig. 2d–h plot the band structures at the five black points in Fig. 2a . We keep the ratio μ 2z /μ 1z =1.76 unchanged and gradually increase μ 2// /μ 1// from 1.1 to 1.4. The irreducible representations of the eigenmodes are labelled to trace the band inversion behaviour. As the ratio μ 2// /μ 1// increases, the two eigenmodes at M point first merge together ( Fig. 2e ) and reopen ( Fig. 2f ), and then the two eigenmodes at K point switch order ( Fig. 2f,h ). In both inversions, the bandgap closes and reopens along with the change of spin Chern number. Furthermore, when μ 2// /μ 1// <1, there are two PTI phases due to the band inversion at K point. Spin Chern numbers of both phases are non-zero, but have opposite signs indicating the opposite propagation directions of their spin-up (spin-down) edge states. In general, topologically protected state supporting robust transport will exist at the boundary separating a PTI and a topologically trivial photonic insulator. We first constructed a flat edge between a PTI and a low-index waveguide which comprises a pair of parallel plates filled with the homogeneous medium of and . The low-index waveguide serves as a trivial photonic insulator below its cutoff frequency of 0.3125 ( c / a ). 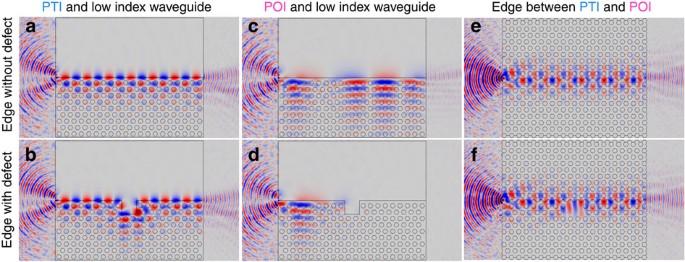Figure 3: Robust transport in the conceptual metacrystal waveguide. Wave transport at the edge with/without defect between (a,b) PTI and the low-index waveguide, (c,d) POI and the low-index waveguide, (e,f) PTI and POI.b,fillustrate that the defect does not introduce backscattering, whiledshows that the defect causes strong backscattering to the extent that there is no transmitted wave. Figure 3a shows the right-going edge state is guided at the edge between the two insulators, when an H z -polarized magnetic dipole is placed at the left of edge. The two domains at the left and right sides of the edge is filled with a dielectric ( ε =13), where the wave can propagate. To demonstrate the topologically protected properties, a square barrier with a material of and is introduced at the edge to probe the wave transport properties in the presence of defects. Figure 3b demonstrated that the wave can go around the barrier and keep moving rightward, and the amplitude of the transmitted wave is the same as the case without the barrier. It is obvious that the edge transport is robust against a barrier with matched ε/μ ratio which cannot couple the two spin states. As a control calculation, the edge between POI and the low-index waveguide is studied in Fig. 3c,d . Here the EM waves experiences strong backscattering and nearly no transmission can be observed after the square barrier is inserted. Topologically protected state can also exist between PTI and POI, as shown in Fig. 3e,f . The defect is introduced by removing five rods near the PTI edge, and the wave can pass through the defect with no backscattering. In the next section, we will employ such kind of defect to experimentally demonstrate the robust transport. Figure 3: Robust transport in the conceptual metacrystal waveguide. Wave transport at the edge with/without defect between ( a , b ) PTI and the low-index waveguide, ( c , d ) POI and the low-index waveguide, ( e , f ) PTI and POI. b , f illustrate that the defect does not introduce backscattering, while d shows that the defect causes strong backscattering to the extent that there is no transmitted wave. Full size image Experimental observation of topological edge states To experimentally realize the PTI, we constructed samples using carefully designed non-resonant meta-atoms ( Fig. 1a ). The meta-atoms have the same ‘gyro’ and ‘star’ geometries, but are arranged in conjugate patterns for POI (upper half in Fig. 1b ) and PTI (lower half in Fig. 1b ) and different geometry dimensions ( Fig. 1c–f ; see Methods). All PTI bands are nearly double degenerate from 1.6 to 3.2 GHz ( Fig. 4b ). A non-trivial bandgap spanning from 2.65 to 2.93 GHz (highlighted by blue color) is achieved. Microwave transmission spectra in Fig. 4a,c confirmed the theory-predicted bandgaps along ΓM and ΓK directions. For the POI ( Fig. 4e ), the photonic bands are almost identical to those of PTI, but with a distinct topological classification from the PTI. 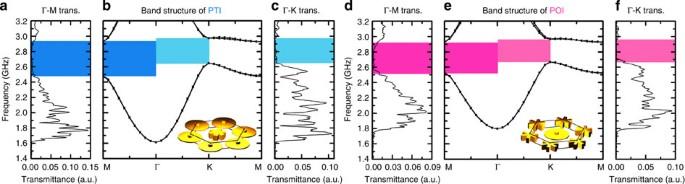Figure 4: Bulk band structures and measured transmissions of PTI and POI. (a,c) Measured transmission spectrum of the PTI along ΓM/ΓK direction. (b) Calculated band structure of the PTI. Black frames in the insets ofb,eoutline the single-layer cell, which is repeated six times in thezdirection. (d–f) Results for POI. Figure 4: Bulk band structures and measured transmissions of PTI and POI. ( a , c ) Measured transmission spectrum of the PTI along ΓM/ΓK direction. ( b ) Calculated band structure of the PTI. Black frames in the insets of b , e outline the single-layer cell, which is repeated six times in the z direction. ( d – f ) Results for POI. Full size image Spin-filtered gapless edge state is a signature feature at the boundary of two ε/μ- matched materials with different topological characters. Such a boundary is realized by placing two metacrystal waveguides side-by-side (green line in Fig. 1a ). 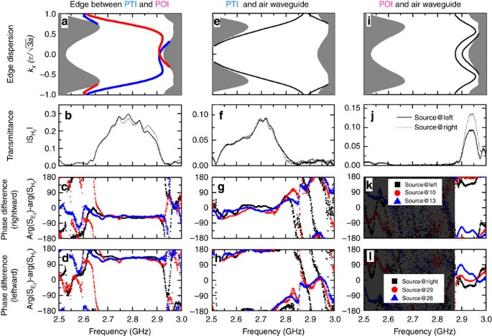Figure 5: Propagation characteristics of the edge states between two photonic insulators. (a) Edge state dispersion for the boundary between PTI and POI. (b) Measured transmissions for the rightward (solid) and leftward (dotted) directions. (c) Phase differences between the Ezand Hzcomponents at the right exit when the source is placed at either the left entrance (black), in the 10th hole (red) or in the 13th hole (blue). An obvious phase plateau at −50° appears in the complete bandgap no matter where the source locates, since only the spin-up rightward state can be detected at the right end. (d) Phase differences between the Ezand Hzcomponents when the exit is on the left and the source is placed at the right entrance (black), in the 29th hole (red) or in the 26th hole (blue). The phase differences stabilize around 130°. Bothc,ddemonstrate the spin-filtered feature of the gapless topological states between PTI and POI. (e–h) results for the edge between PTI and air waveguide. (i–l) results for the edge between POI and air waveguide. Figure 5a shows that the spin-up/down gapless states (blue/red curves) span the whole bandgap and connect to the neighbouring bulk bands (grey areas). The corresponding measured transmission spectra were illustrated in Fig. 5b , where high transmittance occurs within the frequency range of the gapless states. Moreover, the edge in this bandgap is spin-filtered, as the group velocity of spin-up/down state always points to the + x /− x direction. So when the source was at the left, only a rightward spin-up state can be excited, indicating that the E z and H z fields are in phase throughout the upper half of waveguide. As the probe antenna was placed outside the waveguide, the transmitted waves on the exit would acquire additional phases due to different impedances for TE 1 and TM 1 modes. As a result, the measured phase difference (see Methods) between the E z and H z fields of the gapless topological state would be constant but deviate from 0°. This was verified by the phase plateau around −50° from 2.68 to 2.92 GHz (black in Fig. 5c ). In addition, since the spin-up state was the only allowed rightward mode, the phase difference at the right exit should not vary regardless where the source is positioned. This was also demonstrated by the measured phase differences (red and blue curves) in Fig. 5c (see also the transmission coefficients in Supplementary Fig. 5 and Note 4 ). When the source is put into the sample, both rightward spin-up edge state and leftward spin-down edge state can be excited. However, only the spin-up wave can reach the detector because no edge state exists between PTI and air surrounding. For the leftward spin-down state, it could be excited if the source and detector switched positions. Measure transmission was still high (dotted line in Fig. 5b ), and the phase differences at the left exit were stable around 130° independent of source position ( Fig. 5d ). Figure 5: Propagation characteristics of the edge states between two photonic insulators. ( a ) Edge state dispersion for the boundary between PTI and POI. ( b ) Measured transmissions for the rightward (solid) and leftward (dotted) directions. ( c ) Phase differences between the E z and H z components at the right exit when the source is placed at either the left entrance (black), in the 10th hole (red) or in the 13th hole (blue). An obvious phase plateau at −50° appears in the complete bandgap no matter where the source locates, since only the spin-up rightward state can be detected at the right end. ( d ) Phase differences between the E z and H z components when the exit is on the left and the source is placed at the right entrance (black), in the 29th hole (red) or in the 26th hole (blue). The phase differences stabilize around 130°. Both c , d demonstrate the spin-filtered feature of the gapless topological states between PTI and POI. ( e – h ) results for the edge between PTI and air waveguide. ( i – l ) results for the edge between POI and air waveguide. Full size image Propagation characteristics for two other types of boundaries are measured for comparison. The first instance is the boundary between the PTI and air waveguide. The air waveguide can serve as a trivial photonic insulator below the cutoff frequency of 3.125 GHz. The spin-filtered feature can still be maintained in a certain frequency range while the gapless feature is absent (as the air waveguide is not ε/μ matched to PTI). The measured results are shown in Fig. 5g,h that the phase plateau locates around 10° (175°) from 2.65 to 2.75 GHz, when the EM wave propagates from the left (right) side. At the zone boundary, a minigap opens for the ε/μ mismatching between PTI and air waveguide ( Fig. 5e ), leading to low measured transmittances from 2.85 to 2.92 GHz ( Fig. 5f ). The phase differences of the spin state near the minigap deviate from 10° and 175° due to spin mixing. Next we consider the edge between the POI and air waveguide. High transmission can only be observed above 2.87 GHz ( Fig. 5j ), which confirms the existence of gapped edge states (rather than gapless edge states) between two trivial insulators ( Fig. 5i ). In contrast to the PTI case, the phase differences of the edge states no longer stabilize at a certain value, and are dependent on the position of source loop because of the coexistence of multiple edge states ( Fig. 5k,l ). The frequency regions below 2.87 GHz are shaded in Fig. 5k,l as this frequency range do not carry useful information. To demonstrate transport robustness at the boundary between PTI and POI, a defect was introduced inside PTI by substituting five unit cells of ‘star’ meta-atoms by ‘gyro’ meta-atoms near the centre of the edge (dashed panes in Fig. 6a,b ). 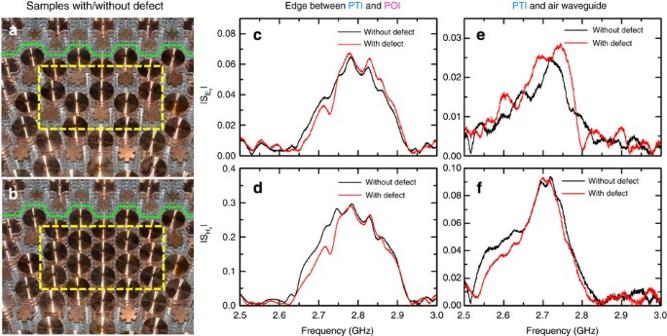Figure 6: Robust transport at the edge of PTI. (a,b) Close-up view of the sample with/without defect. (c,d) Transmission coefficients of the Ez/Hzfield for the edge between PTI and POI. Black is for the case of no defect, while red is for the defect with five unit cells of star meta-atoms being substituted by gyro meta-atoms. The right-going spin-up edge state keeps moving rightward even when it encounters a defect, due to the absence of left-going spin-up edge state. (e,f) Measured transmissions for the edge between PTI and air waveguide. Robust transport can also be observed from 2.65 to 2.75 GHz where spin-filtered feature is maintained. High transmission of the E z and H z fields was maintained even when the defect was present ( Fig 6c,d ). When the right-going spin-up state encountered a defect, it has no choice but to keep moving rightward for the absence of left-going spin-up state. Figure 6e,f plots the transmission coefficients for the edge between PTI and air waveguide with/without defect. It is found that robust transport can also be observed from 2.65 to 2.75 GHz for the spin-filtered feature. Figure 6: Robust transport at the edge of PTI. ( a , b ) Close-up view of the sample with/without defect. ( c , d ) Transmission coefficients of the E z /H z field for the edge between PTI and POI. Black is for the case of no defect, while red is for the defect with five unit cells of star meta-atoms being substituted by gyro meta-atoms. The right-going spin-up edge state keeps moving rightward even when it encounters a defect, due to the absence of left-going spin-up edge state. ( e , f ) Measured transmissions for the edge between PTI and air waveguide. Robust transport can also be observed from 2.65 to 2.75 GHz where spin-filtered feature is maintained. Full size image In summary, we proposed and realized experimentally a PTI by embedding an anisotropic photonic crystal into a metallic plate waveguide. The cross coupling between TE and TM waveguide modes introduces an effective coupling which opens a wide non-trivial bandgap in non-bianisotropic metacrystal with a mild dispersion. Our experimental results confirmed the gapless spin-filtered behaviour and the robust transport expected for PTI. The concept of crystal waveguide in this work can be a useful platform to experimentally investigate photonic topological state. Designs of PTI and POI metacrystal waveguides To experimentally realize the photonic topological states in metacrystal waveguides, we constructed both PTI and POI by non-resonant meta-atoms. The types of meta-atoms in the topologically trivial/non-trivial insulators have the same shape (‘gyro’ and ‘star’) except the conjugate arrangements. For the ‘gyro’ atom, the disc gives a strong diamagnetic response to vertical magnetic field leading to a smaller effective permeability constant in the z direction, that is, μ z <μ // . Meanwhile, the ‘star’ atom can be viewed as three erected slabs each rotated 120° to preserve the C 6 symmetry of the crystal. The erected slabs give a diamagnetic response in the horizontal directions, yielding μ z >μ // . If we want to construct a PTI (inset of Fig. 2a ), we can implement the ‘rod’ using the ‘star’ ( Fig. 1e ) and use the ‘gyro’ ( Fig. 1f ) as the background. We can also construct a POI by filling the rod with ‘gyro’ surrounded by six ‘stars’ ( Fig. 1b ). In addition, the capacitance between neighbouring ‘gyros’ (also between neighbouring ‘stars’) results in a substantial dipole moment, and thus the horizontal and vertical component of the effective permittivity (ε // and ε z ) can be controlled by geometry dimensions of the ‘gyro’ (and ‘star’), to fulfil the ε/μ- matching condition (see Supplementary Fig. 6 and Note 5 ) in the frequency range from 2.5 to 3 GHz due to the non-resonant feature of the meta-atoms. All the simulation results in this paper is calculated by COMSOL Multiphysics. Experimental setup Supplementary Figure 4 shows a detailed experimental setup, where metamaterials are denoted by coloured hexagonal rods for simplicity. The compositions are shown in the dashed panes. In the measurement, we drilled 38 holes on the top copper plate at the edge line, and put the source antenna into the sample. In this way, we can excite the edge states inside the sample, rather than at the left entrance. Only one hole is opened while the other 37 holes are blocked each time. The 10th, 13th, 26th and 29th holes are marked by black arrows. The source antenna is a 12-mm-diameter loop emitted the H z -polarized microwave. It was placed at the left of the edge to excite the rightward edge state. There were two probes, a 24-mm-long monopole antenna and a loop antenna with a diameter of 20 mm, respectively. The monopole antenna was placed in the top half of waveguide to measure the E z field due to the zero node of the E z field at the central plane ( z =24 mm). The probe loop antenna was placed at the central plane for a stronger coupling to the first order waveguide mode. All the probe antennas were positioned 2 cm away from the exit. The four rightmost panels in Supplementary Fig. 4 show how to measure the E z and H z fields. Both fields need to be obtained by measuring twice, respectively. The first and second panels show the antenna positions for the E z field measurement, The monopole antenna was placed at the top half (from z =24 mm to z =48 mm) and then placed upside down at the bottom half (from z =0 mm to z =24 mm). By averaging the two scattering parameters (S E1 and S E2 ), the E z field from TM 0 mode can be cancelled out, and only the E z field from the first order mode was left. The third and fourth panels show the antenna positions for the H z field measurement. If the loop antenna is laid horizontally in the xy plane, it can sense not only the H z field but also the E x and E y fields. To retrieve the H z field, we place the loop with its gap to the right and then rotate the loop by 180° in the xy plane. By averaging the two scattering parameters (S H1 and S H2 ), the electric field components can be eliminated. Finally, the transmission coefficients of the EM wave through the boundary of photonic insulators is equivalent to the average quantities normalized by a linear polarized plane wave propagating in the + x direction. How to cite this article: Chen, W.-J. et al. Experimental realization of photonic topological insulator in a uniaxial metacrystal waveguide. Nat. Commun. 5:5782 doi: 10.1038/ncomms6782 (2014).